METTL3-dependent m6A modification programs T follicular helper cell differentiation T follicular helper (T FH ) cells are specialized effector CD4 + T cells critical to humoral immunity. Whether post-transcriptional regulation has a function in T FH cells is unknown. Here, we show conditional deletion of METTL3 (a methyltransferase catalyzing mRNA N 6 -methyladenosine (m 6 A) modification) in CD4 + T cells impairs T FH differentiation and germinal center responses in a cell-intrinsic manner in mice. METTL3 is necessary for expression of important T FH signature genes, including Tcf7 , Bcl6 , Icos and Cxcr5 and these effects depend on intact methyltransferase activity. m 6 A-miCLIP-seq shows the 3′ UTR of Tcf7 mRNA is subjected to METTL3-dependent m 6 A modification. Loss of METTL3 or mutation of the Tcf7 3′ UTR m 6 A site results in accelerated decay of Tcf7 transcripts. Importantly, ectopic expression of TCF-1 (encoded by Tcf7 ) rectifies T FH defects owing to METTL3 deficiency. Our findings indicate that METTL3 stabilizes Tcf7 transcripts via m 6 A modification to ensure activation of a T FH transcriptional program, indicating a pivotal function of post-transcriptional regulation in promoting T FH cell differentiation. The production of high-affinity antibodies and generation of memory cells are critical for establishing protective immunity [1] , [2] . During acute viral infection, T follicular helper (T FH ) cells provide help to cognate antigen-presenting B cells to facilitate the formation of germinal centers (GCs) and the development of long-lived plasma cells and memory B cells [3] . After priming by dendritic cells (DCs) in the T-cell zone, CD4 + T cells upregulate the expression of chemokine receptor CXCR5, the costimulatory receptor ICOS and the transcriptional repressor B-cell lymphoma 6 (Bcl-6), which together coordinate early fate commitment of T FH cells and their migration to the follicles. After interacting with cognate antigen-presenting B cells, these activated CD4 + T cells mature into T FH cells and further differentiate into GC T FH cells, providing help to GC B cells for humoral immunity [4] , [5] . T FH differentiation is a complicated biological process [6] , which is tightly controlled by multiple transcription factors. As a master regulator of T FH differentiation, Bcl-6 represses the T H 1, T H 2, and T H 17 lineage-specific transcription factors to promote the differentiation of activated CD4 + T cells into T FH cells [7] , [8] , [9] . On the contrary, Blimp1 (encoded by Prdm1 ) negatively modulates Bcl-6 transcription by binding to the Bcl6 promoter and acting as a repressor, thus preventing T FH differentiation and promoting the formation of non-T FH effector helper T cells [9] , [10] . Accumulative studies have demonstrated that TCF-1 (encoded by Tcf7 ) plays key roles in T FH differentiation by directly acting upstream of the Bcl-6–Blimp1 axis [11] , [12] , [13] . Although the regulation of these transcription factors has been intensely investigated at the transcriptional level, it remains unknown if post transcriptional mechanisms are involved in the balanced expression of these key factors during T FH differentiation. N 6 -methyladenosine (m 6 A) is the most prevalent modification on eukaryote mRNAs, catalyzed by m 6 A methyltransferases [14] . Methyltransferase like 3 protein (METTL3, encoded by Mettl3 ) is the core catalytic subunit of m 6 A methyltransferases, and METTL14 is an allosteric activator of METTL3 [15] , [16] . The recruitment of m 6 A-binding proteins is actively involved in almost every stage of mRNA metabolism, from processing in the nucleus to translation and decay in the cytoplasm, adding another layer of regulatory mechanisms in gene expression [17] . Early studies showed that m 6 A-tagged transcripts had shorter half-life [18] , and binding of YTHDF2 to m 6 A promoted m 6 A-modified mRNA decay [18] , [19] . Recently, it was discovered that a group of novel m 6 A-binding proteins, IGF2BPs, stabilized methylated transcripts by guarding them against degradation [20] , [21] . The distinct roles of YTHDF2 and IGF2BPs suggest that the impact of m 6 A modification on mRNA stability is highly dependent on cell context. Several studies have uncovered critical roles of m 6 A modification in immune regulation. It has been documented that m 6 A methylation is essential for normal hematopoiesis and leukemia development [22] , [23] , [24] . m 6 A methylation regulates T-cell homeostasis, as well as suppressive functions of Treg cells by targeting Socs genes [25] , [26] . In the context of viral infection, m 6 A represses type I interferon production in an innate antiviral state [27] , [28] . Despite these profound effects of m 6 A modification on immunoregulation, its role in T FH differentiation has not been determined. In this study, by conditional targeting the Mettl3 gene in T cells, we demonstrate that METTL3-mediated m 6 A modification is critical for T FH cell differentiation. Mechanistically, METTL3 deficiency impairs the stability of m 6 A-modified Tcf7 mRNA, resulting in compromised activation of T FH transcriptional program. METTL3 controls T FH differentiation and GC reactions To investigate the role of METTL3 in T FH differentiation, Mettl3 -floxed mice were crossed with Cd4 -Cre mice to generate conditional deletion of METTL3 in T cells ( Mettl3 fl/fl Cd4 -Cre mice), and the deletion efficiency of METTL3 in splenic CD4 + T cells was validated by quantitative RT-PCR (Supplementary Fig. 1a ). We then infected Mettl3 fl/fl Cd4 -Cre mice and their wild-type control littermates (Ctrl) with LCMV-Armstrong strain. The frequency and numbers of CD44 + CXCR5 + T FH cells were significantly diminished in Mettl3 fl/fl Cd4 -Cre mice compared with those in their control littermates on day 8 post viral infection (Fig. 1a, b ). In contrast, METTL3-deficient CD4 + T cells were dramatically skewed toward the CD44 + CXCR5 − T H 1 proportion, albeit the numbers of T H 1 cells were also decreased with the ablation of METTL3 (Fig. 1a, b ). It is worth mentioning that ablation of METTL3 resulted in more severe defects in T FH cells (21.4-fold change) than T H 1 cells (1.9-fold change) upon acute viral infection (Fig. 1b ). Given T-bet is expressed at a relatively high level on T H 1 lineage and directs its commitment [29] , we also analyzed T-bet expression on both T H 1 and T FH cells. We found T H 1 cells expressed a much higher level of T-bet than T FH cells, and both T FH and T H 1 cells downregulated T-bet expression in the absence of METTL3 (Supplementary Fig. 1b ). Moreover, Mettl3 fl/fl Cd4 -Cre mice exhibited remarkably lower percentages and absolute cell numbers of GC T FH cells (identified as PD-1 hi CXCR5 + , ICOS hi CXCR5 + , or Bcl-6 hi CXCR5 + ) than those of their control littermates (Fig. 1c, d ). Accordingly, the expression levels of CXCR5, PD-1, ICOS, and Bcl-6 were dramatically lower on METTL3-deficient T FH cells than on wild-type cells (Supplementary Fig. 1c, d ). These results indicated that METTL3 deficiency severely impairs T FH differentiation. Fig. 1: Conditional ablation of METTL3 impairs T FH differentiation and GC responses. a , b Flow cytometry analysis of CD44 + CXCR5 + T FH cells and CD44 + CXCR5 – T H 1 cells, gated on splenic CD4 + T cells from Ctrl and Mettl3 fl/fl Cd4 -Cre mice on day 8 post infection (8 dpi ). Summary of the frequency and cell numbers of indicated cell subsets are shown in b ( n = 5 per group). c , d Flow cytometry analysis of PD-1 hi CXCR5 + GC T FH cells (top panel), ICOS hi CXCR5 + GC T FH cells (middle panel), and Bcl-6 hi CXCR5 + GC T FH cells (bottom panel), gated on splenic CD44 hi CD62L lo CD4 + T cells from Ctrl and Mettl3 fl/fl Cd4 -Cre mice on 8 dpi . Summary of the frequency and cell numbers of indicated cell subsets are shown in d ( n = 5 per group). e , f Flow cytometry analysis of splenic GL-7 + Fas + GC B cells (top panel) and IgD lo CD138 + plasma cells (bottom panel) on 8 dpi . Summary of the frequency and cell numbers of GC B cells and plasma cells are shown in f ( n = 3 per group). g Immunofluorescent staining of spleens from Ctrl and Mettl3 fl/fl Cd4 -Cre on 8 dpi . Green: PNA; Red: IgD; scale bar: 10 μm. h Analysis of LCMV-specific IgG concentration in serum on 8 dpi (top) and on 56 dpi (bottom) by ELISA (day 8: n = 12 for Ctrl group, n = 10 for Mettl3 fl/fl Cd4 -Cre group; day 56: n = 5 per group). Data are representative of at least three independent experiments. Error bars indicate standard error of the mean. P value was calculated by unpaired two-tailed Student’s t test. Full size image Given the main function of T FH cells is to provide cognate B-cell help, which is a fundamental aspect of humoral immunity and generation of immunological memory [1] . We next examined whether METTL3 deficiency in CD4 + T cells affects GC formation during viral infection. A robust reduction in the proportions and numbers of GL-7 + Fas + GC B cells (Fig. 1e, f ) and PNA + Fas + GC B cells (Supplementary Fig. 1e, f ) were observed in Mettl3 fl/fl Cd4 -Cre mice, compared with those in their wild-type counterparts. Furthermore, the frequency and cell numbers of IgD lo CD138 + plasma cells were also much lower in Mettl3 fl/fl Cd4 -Cre mice than those in wild-type mice (Fig. 1e, f ). The immunohistochemical analysis further confirmed substantially reduced PNA + GCs within B-cell follicles in spleens from Mettl3 fl/fl Cd4 -Cre mice (Fig. 1g ). To assess the consequences of defective T FH and GC responses in Mettl3 fl/fl Cd4 -Cre mice, we measured the LCMV-specific serum concentration of immunoglobulin G (IgG). The LCMV-specific IgG concentration was significantly lower in Mettl3 fl/fl Cd4 -Cre mice than that in their wild-type control littermates on day 8 and day 56 post viral infection (Fig. 1h ). Collectively, these results suggested that METTL3 is required for T FH differentiation and GC responses. To further validate these findings, we immunized Mettl3 fl/fl Cd4 -Cre mice and their wild-type control littermates by intraperitoneal administration of keyhole limpet hemocyanin (KLH) emulsified in Complete Freund’s Adjuvant (CFA). On day 8 post immunization, Mettl3 fl/fl Cd4 -Cre mice exhibited impaired development of T FH cells and GC T FH cells, but not T H 1 cells (Supplementary Fig. 2a, b ). Meanwhile, the percentages and cell numbers of GC B cells and plasma cells (Supplementary Fig. 2c, d ) were also impaired in Mettl3 fl/fl Cd4 -Cre mice compared with their wild-type counterparts. These data jointly indicated METTL3 promotes T FH differentiation upon different antigen stimulation. Meanwhile, the differentiation of other T helper lineages was also examined by using KLH immunization model. We found that both GATA3 + and IL-4-producing cells, as well as Foxp3 + cells were not altered in Mettl3 fl/fl Cd4 -Cre mice (Supplementary Fig. 2e–h ), indicating T H 2 and Treg cell differentiation are not affected in the absence of METTL3 upon KLH immunization. Interestingly, both RORγt + and IL-17a-producing cells were significantly decreased in METTL3-deficient mice (Supplementary Fig. 2e–h ), revealing METTL3 is essential for T H 17 cell differentiation in vivo upon protein immunization. METTL3 intrinsically regulates T FH differentiation We next focused on whether METTL3 regulates T FH differentiation in a cell-intrinsic manner using both bone marrow chimeric and adoptive transfer mice models. We first generated bone marrow chimeric mice by reconstituting lethally irradiated wild-type recipient mice (CD45.1 + ) with a mixture donor of bone marrow cells from Mettl3 fl/fl Cd4 -Cre mice (CD45.2 + ) and wild-type (CD45.1 + ) competitor mice (Supplementary Fig. 3a ). On day 8 post LCMV-Armstrong infection, Mettl3 fl/fl Cd4 -Cre mice-derived CD4 + T cells had much lower cell numbers of CD44 + CXCR5 + T FH cells than those of competitor bone marrow-derived CD4 + T cells (Supplementary Fig. 3b, c ). Correspondingly, CD4 + T cells originated in Mettl3 fl/fl Cd4 -Cre mice also exhibited a reduction of PD-1 hi CXCR5 + GC T FH cells (Supplementary Fig. 3b, c ). The expression levels of CXCR5, PD-1, ICOS, and Bcl-6 were significantly lower on METTL3-deficient T FH cells than those on competitor cells (Supplementary Fig. 3d ). To further rule out the effect of external factors on T FH differentiation, we adoptively transferred CD45.1 + SMARTA CD4 + T cells into CD45.2 + Mettl3 fl/fl Cd4 -Cre or their wild-type control littermates (Fig. 2a ). On day 8 post viral infection, we observed the percentages and numbers of CD44 + CXCR5 + T FH cells derived from CD45.1 + SMARTA CD4 + T cells were similar in the Mettl3 fl/fl Cd4 -Cre mice and their wild-type counterparts (Fig. 2b, c ), indicating the microenvironment in the Mettl3 fl/fl Cd4 -Cre mice did not impair T FH differentiation. In contrast, METTL3-deficient CD4 + T cells displayed compromised T FH differentiation compared with that of congenic wild-type CD4 + T cells (Fig. 2b, c ). Correspondingly, METTL3-deficient CD4 + T cells also exhibited defects in their ability to differentiate into CD44 + CXCR5 − T H 1 cells (Fig. 2b, c ). Besides, transferred CD45.1 + SMARTA cells also profoundly promoted the GC B and plasma cells differentiation (Fig. 2d, e ), GC formation (Fig. 2f ), and excessive production of LCMV-specific IgG antibody (Fig. 2g ) in Mettl3 fl/fl Cd4 -Cre recipients. Together, our data demonstrated METTL3 is intrinsically required for T FH cell differentiation and functions as a key role in GCs formation. Fig. 2: METTL3 intrinsically controls T FH differentiation and GC responses. a Scheme of adoptive transfer model. 5 × 10 6 CD45.1 + SMARTA cells were adoptively transferred into CD45.2 + Mettl3 fl/fl Cd4 -Cre mice or Ctrl host mice, followed by LCMV-Armstrong infection within 24 h. b , c Flow cytometry analysis of CD45.1 + SMARTA or CD45.2 + host T cell-derived CD44 + CXCR5 + T FH and CD44 + CXCR5 – T H 1 cells, gated on splenic CD4 + T cells from host mice on day 8 post viral infection. Frequency and numbers of CD44 + CXCR5 + T FH cells and CD44 + CXCR5 – T H 1 cells are shown in c ( n = 5 per group). d , e Flow cytometry analysis of splenic PNA + Fas + GC B cells (top panel) and IgD lo CD138 + plasma cells (bottom panel) from host mice on 8 dpi . Summary of the frequency and cell numbers of GC B cells and plasma cells are shown in e ( n = 6 per group). f Immunofluorescent staining of spleens from Ctrl or Mettl3 fl/fl Cd4 -Cre host mice on 8 dpi . Green: PNA; Red: IgD; scale bar: 10 μm. g Analysis of LCMV-specific IgG concentration in serum on 8 dpi by ELISA ( n = 5 for Ctrl group, n = 5 for Mettl3 fl/fl Cd4 -Cre group, n = 6 for Ctrl host group, n = 6 for Mettl3 fl/fl Cd4 -Cre host group). Data are representative of at least three independent experiments. Error bars indicate standard error of the mean. P value was calculated by unpaired two-tailed Student’s t test ( e ) or two-way ANOVA coupled with multiple comparisons ( c , g ). Full size image METTL3 is essential for the early initiation of T FH cells During acute viral infection, effector CD4 + T cells’ commitment to the T FH lineage or T H 1 lineage emerges before the initiation of GCs [12] . To investigate whether METTL3 is required for early T FH specification in vivo, naive Ctrl or Mettl3 fl/fl Cd4 -Cre SMARTA CD4 + T cells were labeled with cell-trace violet (CTV) and adoptively transferred into congenic recipient mice, followed by LCMV-Armstrong infection (Supplementary Fig. 4a ). On day 3 post viral infection, SMARTA CD4 + T cells of both genotypes showed similar upregulation of T-cell activation markers CD69 and CD44, and downregulation of CD62L (Supplementary Fig. 4b, c ). In vitro cell culture analysis also revealed that Mettl3 fl/fl Cd4 -Cre SMARTA CD4 + T cells displayed no obvious defects in T-cell activation (Supplementary Fig. 4d ). Ctrl SMARTA CD4 + T cells exhibited vigorously proliferation post viral infection, whereas METTL3-deficient cells displayed a delayed proliferation (Fig. 3a ). Lineage commitment to T FH lineage has occurred on day 3 post viral infection, as detected by Bcl-6 + CXCR5 + cells [30] . Consistently, wild-type SMARTA cells developed robust numbers of Bcl-6 + CXCR5 + T FH cells, whereas METTL3-deficient cells exhibited much lower percentages and cell numbers of Bcl-6 + CXCR5 + T FH cells (Fig. 3b ). Tracking the cell division showed Mettl3 fl/fl Cd4 -Cre SMARTA cells were predominantly in third and fourth divisions, while Ctrl SMARTA cells had advanced to fifth and sixth divisions (Fig. 3c, d ), reflecting the impaired proliferation of activated CD4 + T cells in the absence of METTL3. Consistently, Mettl3 fl/fl Cd4 -Cre SMARTA cells exhibited a reduction of proportions and cell numbers of Bcl-6 + CXCR5 + T FH cells in indicated cell divisions compared with that of Ctrl SMARTA cells (Fig. 3e, f ). Interestingly, as a critical regulator for early T FH differentiation [31] , TCF-1 expression in CXCR5 + cells was also dramatically reduced due to ablation of METTL3 (Fig. 3g, h ). Moreover, we also observed compromised CD25 − CXCR5 + T FH cells in Mettl3 fl/fl Cd4 -Cre SMARTA cells by using the combination of CXCR5 and CD25 to identify T FH cells in activated CD4 + T cells (Supplementary Fig. 4e, f ), and apoptosis of T FH cells was elevated in the absence of METTL3 (Supplementary Fig. 4g, h ). We further assessed the expression levels of genes that are associated with T FH cells, including Tcf7 , Cxcr5 , Bcl6 , Pdcd1 , and Icos . The expression levels of these genes were substantially decreased in Mettl3 fl/fl Cd4 -Cre SMARTA T FH cells compared with those of Ctrl cells (Fig. 3i ). Correspondingly, the expressions of Prdm1 and Id2 , both well-known for promoting T H 1 differentiation [9] , [32] , were much lower in Ctrl T FH cells than that of Mettl3 fl/fl Cd4 -Cre SMARTA cells (Fig. 3i ). These results thus demonstrated that METTL3 is indispensable for early T FH commitment during acute viral infection. Fig. 3: METTL3 is indispensable for the initiation of T FH development. a Flow cytometry analysis of cells from the wild-type recipient mice (CD45.1 + ) given adoptive transfer of naive CTV-labeled Ctrl or Mettl3 fl/fl Cd4 -Cre SMARTA cells, followed by LCMV-Armstrong infection and analysis 3 days later as CTV dilution by the transferred cells. b Flow cytometry analysis of Bcl-6 + CXCR5 + T FH cells gated on SMARTA CD4 + T cells from recipient mice as in a . Summary of the frequency and cell numbers of T FH cells are shown on the right ( n = 3 per group). c , d Flow cytometry analysis of different cell divisions gated on SMARTA CD4 + T cells from recipient mice as in a . The frequency of third to sixth divisions is summarized in d ( n = 3 per group). e , f Contour plots display Bcl-6 + CXCR5 + T FH cells in indicated divisions, among SMARTA cells from recipient mice as in a . Summary of the frequency and cell numbers of T FH cells in indicated divisions are shown in f ( n = 3 per group). g , h Flow cytometry analysis of the expression of TCF-1 in CXCR5 + cells in indicated divisions gated on SMARTA CD4 + T cells from recipient mice as in a . Quantification of geometric mean fluorescence intensity (gMFI) of TCF-1 in indicated divisions is shown in h ( n = 3 per group). i Quantitative RT-PCR analysis of mRNA abundance of T FH cell-related genes in CD25 – CXCR5 + T FH cells from recipient mice as in a , relative expression was normalized to Ctrl cells ( n = 6 per group). Data are representative of two independent experiments. Error bars indicate standard error of the mean. P value was calculated by unpaired two-tailed Student’s t test ( b , i ) or two-way ANOVA coupled with multiple comparisons ( f , h ). Full size image METTL3 orchestrates the transcriptional profiles of T FH cells We next investigated how METTL3 deficiency affects the transcriptional profiles of T FH cells. Considering CD4 + T cells generally differentiate into T H 1 cells or T FH cells upon acute viral infection [33] and METTL3 deficiency affects CXCR5 expression, we hence used CD44 and SLAM, which is expressed at low level on T FH cells [9] , to identify T H 1 and T FH cells in activated CD4 + T cells. CD44 + SLAM hi T H 1 cells and CD44 + SLAM lo T FH cells were sorted from Mettl3 fl/fl Cd4 -Cre mice and their Ctrl littermates on day 8 post viral infection and subjected to RNA-seq analysis. Compared with those in wild-type cells, 515 upregulated genes and 252 downregulated genes in METTL3-deficient T FH cells (Fig. 4a ) and 763 upregulated genes and 332 downregulated genes (Supplementary Fig. 5a ) in METTL3-deficient T H 1 cells were identified, respectively (≥2-fold expression change, adjusted P value <0.01). In particular, the upregulated genes in T FH cells were significantly enriched in the T-cell differentiation and defense response to virus; the downregulated genes in T FH cells were apparently enriched in T-cell proliferation and differentiation (Fig. 4b ). Then we selected a T FH cell and a GC T FH cell signature gene set [11] for gene set enrichment analysis (GSEA). Both the T FH lineage gene set and the GC T FH -associated gene set were enriched in wild-type T FH cells, but not in METTL3-deficient T FH cells (Fig. 4c ). When applying GSEA to exhibit the signature genes of T H 1 (ref. [12] ), T H 2 (ref. [34] ), T H 17 (ref. [35] ), and Treg [34] cells, we found that all of which were enriched in METTL3-deficient T FH cells (Supplementary Fig. 5b ). Similarly, we also observed T FH , T H 2, T H 17, and Treg-related gene sets were positively enriched in METTL3-deficient T H 1 cells (Supplementary Fig. 5c ). These analyses indicated that loss of METTL3 leads to disordered gene profiles of both T FH and T H 1 transcription program. Fig. 4: Alternation of transcriptional profiles in METTL3-null T FH cells. a Volcano map depicting genes upregulated (red) or downregulated (blue) 2-fold or more in T FH cells on 8 dpi . Heatmap of differentially expressed genes is shown on the right. b Gene Ontology (GO) terms of the differentially expressed genes in Mettl3 fl/fl Cd4 -Cre T FH cells compared with Ctrl T FH cells (Upregulated: top panel; Downregulated: bottom panel). c Gene set enrichment analysis (GSEA) of T FH and GC T FH gene set in Mettl3 fl/fl Cd4 -Cre T FH cells relative to expression in Ctrl T FH cells as in a . d GSEA analysis of “TCF-1-activated genes in T FH cells” and “TCF-1-suppressed genes in T FH cells” (GSE65693) in Mettl3 fl/fl Cd4 -Cre T FH cells relative to expression in Ctrl T FH cells as in a . Heatmaps representation of top 30 ranking genes in the leading edge are shown, respectively. e Quantitative RT-PCR analysis of selected interested genes in a , relative expression was normalized to that in Ctrl T FH cells ( n = 7 for Ctrl group, n = 8 for Mettl3 fl/fl Cd4 -Cre group except Bcl6 gene ( n = 7 per group)). Data are from one experiment with triplicates ( a – d ) or pooled from two experiments ( e ). Error bars indicate standard error of the mean. P value was calculated by unpaired two-tailed Student’s t test ( e ). Full size image We next validated expression changes of key T FH genes and found that Cxcr5 , Bcl6 , Pdcd1 , and Icos were significantly lower in METTL3-null T FH cells than in wild-type cells (Fig. 4e ). In addition, the expression of Tcf7 was lower in METTL3-deficient T FH cells than in wild-type T FH cells (Fig. 4e ). Among the genes with low expression, Tcf7 was of interest because of its role in Tfh cell differentiation, so we also performed GSEA analysis of a gene set containing TCF-1-activated genes in T FH cells [13] . Interestingly, remarkable enrichment was exhibited in wild-type T FH cells, whereas the TCF-1-suppressed gene set [13] was notably enriched in METTL3-deficient cells, which suggested that METTL3 and TCF-1 share a common subset of target genes in T FH cells (Fig. 4d ). Meanwhile, the expression of Lef1 mRNA was also decreased in METTL3-deficient T FH cells compared with wild-type cells (Fig. 4e ). On the other hand, the expression of Prdm1 , known as the antagonist of Bcl6 , and Gzmb was higher in METTL3-null T FH cells than that in wild-type T FH cells (Fig. 4e ). The expression levels of Bcl2l11 and Bax , both known as pro-apoptotic regulators [36] , [37] , were significantly elevated in METTL3-null T FH cells compared with those in the wild-type T FH cells (Fig. 4e ), which corresponded to accelerated apoptosis in Mettl3 fl/fl Cd4 -Cre T FH cells (Supplementary Fig. 4g, h ). In addition, the transcripts encoding other essential transcription factors, receptors and ligands for T FH differentiation, including Batf , Slamf6 , and Il6ra , were downregulated in Mettl3 fl/fl Cd4 -Cre T FH cells compared with those in wild-type cells (Fig. 4e ). Besides, we observed elevated expression of Socs1 mRNA, a known target of METTL3 [25] , [26] , in Mettl3 fl/fl Cd4 -Cre T FH cells (Fig. 4e ). Collectively, these results suggested that METTL3 regulates T FH differentiation program by activating T FH program but suppressing T H 1 lineage-associated genes. METTL3 promotes T FH differentiation in an m 6 A catalytic activity-dependent manner m 6 A methylation is catalyzed by a multicomponent methyltransferase complex, while METTL3 functions as the predominant catalytic subunit [15] , [16] . Next, we analyzed whether METTL3-mediated T FH differentiation is dependent on its m 6 A methyltransferase activity. To achieve this goal, we generated wild-type METTL3 (Mettl3-WT) and catalytic domain mutant METTL3 (D395A and W398A; Mettl3-Mut) constructs [15] (Fig. 5a ). These METTL3 proteins were then expressed in Mettl3 fl/fl Cd4 -Cre SMARTA CD4 + T cells with a retrovirus transduction system (Fig. 5b ). On day 5 post infection, forced expression of Mettl3-WT and Mettl3-Mut both resulted in elevated METTL3 expression in Mettl3 fl/fl Cd4 -Cre SMARTA cells compared with the empty-vector (EV) retrovirus (Fig. 5c ). EV retrovirus-infected Mettl3 fl/fl Cd4 -Cre SMARTA CD4 + T cells exhibited reduced expansion than EV retrovirus-infected Ctrl cells, which could be restored by overexpression of Mettl3-WT but not Mettl3-Mut (Fig. 5d ). Moreover, EV retrovirus-infected Mettl3 fl/fl Cd4 -Cre SMARTA CD4 + T cells remained defective in the generation of CD44 + CXCR5 + T FH cells, while Mettl3-WT but not Mettl3-Mut retrovirus promoted differentiation of Mettl3 fl/fl Cd4 -Cre SMARTA CD4 + T cells into a T FH fate (Fig. 5e ). In addition, forced expression of Mettl3-WT could restore both the cell numbers of Mettl3 fl/fl Cd4 -Cre T FH cells and T H 1 cells (Fig. 5f ). Accordingly, ectopic expression of Mettl3-WT could largely rectify defective PD-1 hi CXCR5 + GC T FH cells in METTL3-deficient cells (Fig. 5g, h ). We also observed that the expression of T FH cell-related genes, including Cxcr5 , Tcf7 , Bcl6 , Pdcd1 , and Icos , were restored in Mettl3 fl/fl Cd4 -Cre cells with inducing Mettl3-WT expression (Fig. 5i ). The data collectively indicated that the m 6 A-catalytic activity of METTL3 is necessary for T FH differentiation. Fig. 5: METTL3 promotes T FH differentiation in an m 6 A catalytic activity-dependent manner. a Graphic representation of the wild-type (Mettl3-WT) and catalytic domain dead (Mettl3-Mut; DPPW to APPA) METTL3 constructs. b Scheme of retrovirus transduction experiment. SMARTA cells were transduced with indicated structures by using a retrovirus transduction system. Then, the transduced cells were adoptively transferred into congenic CD45.2 + wild-type mice followed by LCMV-Armstrong infection, and analyzed on day 5 post viral infection. c Flow cytometry analysis of METTL3 gMFI in GFP + CD4 + SMARTA cells from recipient mice. Quantitation of METTL3 gMFI is shown on the right ( n = 3 per group). d Summary of the frequency and cell numbers of retrovirus-transduced SMARTA CD4 + T cells in host mice ( n = 3 per group). e , f Flow cytometry analysis of CD44 + CXCR5 + T FH populations and CD44 + CXCR5 – T H 1 subsets gated on SMARTA GFP + CD4 + T cells from host mice adoptively transferred with empty vector (EV), Mettl3-WT, or Mettl3-Mut retrovirus-introduced SMARTA cells. Summary of the frequency and cell numbers of T FH cells and T H 1 cells are shown in f ( n = 3 per group). g , h Flow cytometry analysis of PD-1 hi CXCR5 + GC T FH populations gated on SMARTA GFP + CD4 + T cells from host mice adoptively transferred with EV, Mettl3-WT, or Mettl3-Mut retrovirus-introduced SMARTA cells. Summary of the frequency and cell numbers of GC T FH cells are shown in h ( n = 3 per group). i Quantitative RT-PCR analysis of mRNA abundance of T FH cell-related genes in CD44 + CXCR5 + T FH cells ectopically expressed with EV, Mettl3-WT, or Mettl3-Mut, relative expression was normalized to Ctrl cells transduced with EV retrovirus ( n = 6 for Ctrl EV, Mettl3 fl/fl Cd4 -Cre-EV, and Mettl3 fl/fl Cd4 -Cre-Mettl3 WT group; n = 5 for Mettl3 fl/fl Cd4 -Cre-Mettl3 Mut group). Data are representative of two independent experiments. Error bars indicate standard error of the mean. P value was calculated by one-way ANOVA, followed by unpaired two-tailed Student’s t test for indicated pairwise comparisons. Full size image m 6 A modifies Tcf7 mRNA in 3′ UTR to control its stability To examine how m 6 A methylation modulates T FH transcriptional program, we performed m 6 A-miCLIP-SMARTer-seq to map global m 6 A landscape in Ctrl or Mettl3 fl/fl Cd4 -Cre SMARTA CD4 + T cells primed in vivo. Bioinformatic analysis revealed that m 6 A peaks were significantly abundant in 3′ UTR and near the stop codon of mRNAs (Fig. 6a, b ). Approximately 45.3% methylated mRNAs contained three or more peaks (Fig. 6c ). Biological duplicates of m 6 A-miCLIP-SMARTer-seq yielded about 4939 transcripts (called ‘m 6 A-modified transcripts’ hereafter; Fig. 6d ). By stratifying m 6 A-modified transcripts with differentially expressed genes, we found that 208 differentially expressed transcripts were potentially regulated by m 6 A methylation (Fig. 6d ). GO term analysis showed these transcripts were enriched for functions related to defense response to the virus, T-cell activation and differentiation (Fig. 6e ). Among these potential m 6 A methylated target genes, a set of T FH cell-relevant genes were directly marked by m 6 A, such as Cxcr5 , Icos , Il6ra , and Il6st (Supplementary Fig. 6a ). Interestingly, the 3′ UTR of Tcf7 mRNA had highly enriched m 6 A peaks, whereas Bcl6 and Prdm1 mRNAs were not tagged by m 6 A (Fig. 6f and Supplementary Fig. 6a ). Accordingly, RNA immunoprecipitation (RIP) assay suggested METTL3 directly binds to Tcf7 mRNA (Fig. 6g ). The m 6 A-RIP-qPCR results further indicated Tcf7 mRNA was tagged by m 6 A methylation and the m 6 A levels on Tcf7 mRNA were substantially decreased in METTL3-deficient cells (Fig. 6f, h ). These data jointly indicated Tcf7 is a bona fide m 6 A target. Accordingly, both the Tcf7 mRNA and the TCF-1 protein were significantly decreased in METTL3-deficient T FH cells compared with those in wild-type T FH cells (Fig. 4e and Fig. 6i ). To further validate METTL3 regulation of Tcf7 expression in an m 6 A-dependent manner, we identified a high-confidence m 6 A site (GGA 1011 CT, a conserved m 6 A methylation motif) in the Tcf7 3′ UTR region (Fig. 6f ). We generated a minigene vector placing the Tcf7 m 6 A site to the 3′ end of luciferase reporter cDNA. Then the ‘GGACT’ consensus motif in the Tcf7 m 6 A site was mutated into ‘GGTCT’ to abrogate m 6 A modification (Fig. 6j ). Wild-type Tcf7 3′ UTR exhibited increased luciferase activity compared to that of the empty vector (pGL4.23) in the presence of overexpressed METTL3; notably, mutation of Tcf7 3′ UTR almost completely compromised the increase (Fig. 6k ). These results revealed that METTL3 regulates Tcf7 mRNA levels via m 6 A modifications in the 3′ UTR region (m 6 A 1011 ). Given m 6 A modification regulates gene expression by multiple approaches, including mRNA splicing, stability, and translation [17] , [38] , alternative splicing assay was applied and exhibited no significant difference in the alternative splicing of Tcf7 mRNA between Ctrl and METTL3-deficient T FH cells (Supplementary Fig. 6b ). We then performed RNA decay assay via actinomycin D (ActD) treatment to detect the stability of Tcf7 mRNA, and found that Tcf7 mRNA exhibited substantially accelerated decline in METTL3-deficient cells compared with Ctrl cells at checkpoints after treatment (Fig. 6l, m ). Taken together, these data suggested that METTL3 enhances Tcf7 mRNA stability via catalyzing m 6 A methylation at its 3′ UTR, to ensure TCF-1 expression in promoting T FH differentiation. Fig. 6: m 6 A modifies Tcf7 mRNA to control its stability. a Metagene profiles of m 6 A site distribution along a normalized transcript containing three rescaled non-overlapping segments: 5′ UTR, CDS, and 3′ UTR in Ctrl and Mettl3 fl/fl Cd4 -Cre SMARTA CD4 + T cells. b Pie chart showing the distribution of m 6 A sites in five regions of Ctrl and Mettl3 fl/fl Cd4 -Cre SMARTA CD4 + T cells. c Bar chart depicting percentage of mRNAs with different internal m 6 A abundance. d Venn diagram showing the overlapping differentially expressed genes from RNA-seq and m 6 A-modified transcripts from m 6 A-miCLIP-SMARTer-seq. Heatmap of 208 differentially expressed genes with m 6 A modification is shown on the right. e Representative GO terms of the biological process categories enriched in differentially expressed transcripts with m 6 A peaks (Red: upregulated genes; blue: downregulated genes; gray: GO terms). f Integrative Genomics Viewer (IGV) tracks displaying RNA-seq (top panel) and m 6 A-miCLIP-SMARTer-seq (bottom panel) reads distribution of Tcf7 gene. The high-confidence m 6 A site is marked as a triangle. g RIP-qPCR analysis showing enrichment of METTL3 on Tcf7 mRNA in SMARTA CD4 + T cells. The Tcf7 mRNA enrichment is presented as IP/input and normalized to IgG group ( n = 4 per group). h m 6 A-RIP-qPCR analysis of m 6 A enrichment on Tcf7 mRNA of Ctrl and Mettl3 fl/fl Cd4 -Cre SMARTA CD4 + T cells ( n = 4 per group). i Flow cytometry analysis of expression level of TCF-1 on T FH cells on 8 dpi . Quantification of gMFI of TCF-1 is shown on the right ( n = 5 per group). j Constructions of plasmids with wild-type or m 6 A site mutant in Tcf7 3′ UTR. k Luciferase reporter assay. Results were normalized to the luciferase activity of cells co-transfected with the pGL4.23 empty plasmid and EV-Myc plasmid ( n = 6 per group). l RNA decay assay. The half-live of Tcf7 mRNA was detected by quantitative RT-PCR. The remaining mRNAs were normalized to t = 0 ( n = 4 per group). m Quantitative RT-PCR analysis of Tcf7 mRNA abundance as in l , relative expression was normalized to t = 0 of Ctrl cells ( n = 4 per group). Data are from one experiment with duplicate ( a – e ) or representative of at least three independent experiments ( i – h , k – m ). Error bars indicate standard error of the mean. P value was calculated by unpaired two-tailed Student’s t test ( g – i ) or two-way ANOVA coupled with multiple comparisons ( k , m ). Full size image Forced expression of TCF-1 restores defective T FH differentiation in METTL3-deficient mice To determine the functional link between METTL3 and Tcf7 transcript stability in T FH differentiation, we next examined the impact of ectopic expression of TCF-1 in METTL3-deficient cells. Upon transducing in vivo primed SMARTA CD4 + T cells with TCF-1 (full-length CDS of P45 isoform without 3′ untranslated region [39] ) retrovirus (Fig. 7a ), on day 8 post LCMV-Armstrong infection, we observed a significant increase in TCF-1 expression in METTL3-deficient SMARTA cells (Fig. 7b ). We then analyzed T FH populations from transduced SMARTA CD4 + T cells in recipient mice. Compared with Ctrl SMARTA CD4 + T cells infected with EV retrovirus, the EV-infected Mettl3 fl/fl Cd4 -Cre SMARTA CD4 + T cells exhibited defects in CD44 + CXCR5 + T FH differentiation; whereas TCF-1 retrovirus could largely rectify the ability of Mettl3 fl/fl Cd4 -Cre SMARTA CD4 + T cells to differentiate into T FH cells (Fig. 7c ). In addition, TCF-1 overexpression also elevated the cell numbers of Mettl3 fl/fl Cd4 -Cre T FH cells, but not T H 1 cells (Fig. 7d ). Consistently, PD-1 hi CXCR5 + GC T FH cells could also be rescued with TCF-1 overexpression (Fig. 7e, f ). Meanwhile, forced expression of TCF-1 could largely restore the expression levels of TCF-1, CXCR5, PD-1, ICOS, and Bcl-6 on Mettl3 fl/fl Cd4 -Cre T FH cells (Fig. 7g, h ). These data collectively demonstrated that METTL3 stabilizes Tcf7 mRNA expression to promote T FH differentiation. Fig. 7: Enhanced TCF-1 expression rectifies defective T FH differentiation in METTL3-null cell. a Scheme of TCF-1 rescue experiment. SMARTA cells were transduced with TCF-1 structure (full-length CDS of P45 isoform without 3′ UTR region) by using a retrovirus transduction system. Then, the transduced cells were adoptively transferred into congenic CD45.1 + wild-type mice followed by LCMV-Armstrong infection, and analyzed on day 8 post viral infection. b Flow cytometry analysis of TCF-1 gMFI in SMARTA GFP + CD4 + cells from recipient mice on 8 dpi . Quantitation of TCF-1 gMFI is shown on the right ( n = 3 per group). c , d Flow cytometry analysis of CD44 + CXCR5 + T FH populations and CD44 + CXCR5 – T H 1 subsets gated on SMARTA GFP + CD4 + T cells from different host mice adoptively transferred with empty vector (EV) or TCF-1 retrovirus-introduced SMARTA cells at 8 days post infection. Summary of the frequency and cell numbers of T FH cells and T H 1 cells are shown in d ( n = 3 per group). e , f Flow cytometry analysis of PD-1 hi CXCR5 + GC T FH populations gated on SMARTA GFP + CD4 + T cells from different host mice adoptively transferred with EV or TCF-1 retrovirus-introduced SMARTA cells. Summary of the frequency and cell numbers of GC T FH cells are shown in f ( n = 3 per group). g , h Flow cytometry analysis of gMFIs of TCF-1, CXCR5, PD-1, ICOS, and Bcl-6 on CD44 + CXCR5 + T FH cells transduced with EV or TCF-1 retrovirus. Quantification of the gMFIs is shown in h ( n = 3 per group). Data are representative of three independent experiments. Error bars indicate standard error of the mean. P value was calculated by one-way ANOVA, followed by unpaired two-tailed Student’s t test for indicated pairwise comparisons. Full size image N 6 -methyladenosine (m 6 A) accounts for the prevalent mRNA modifications and has recently emerged as a critical epitranscriptomic regulator to affect the translation and stability of the modified transcripts. Here, we showed that ablation of METTL3 leads to substantial defects in both T FH and T H 1 differentiation upon LCMV-Armstrong and KLH challenges. Based on our results, a more severe phenotype was exhibited in T FH cells than that of T H 1 cells from METTL3-deficient mice, which strongly supports the notion that the METTL3 acts as an intrinsic modulator of T FH cells. During acute viral infection, bifurcation of effector CD4 + T cells into T FH cells or T H 1 cells can be observed as early as the second to third division [40] . A recent report demonstrated that METTL3-null CD4 + T cells remained naive state and exhibited defective proliferation when tested both in vivo and in vitro [25] . Using an adoptive transfer model, we found that METTL3-deficient CD4 + T cells showed a delayed differentiation and a slower proliferation upon acute viral infection, although they were activated normally as shown by expression of the surface markers via both in vivo and in vitro assay. Meanwhile, at 72 h post infection, the activated CD4 + T cells were mostly in the fifth and sixth divisions, whereas METTL3-deficient CD4 + T cells were dominant in third and fourth divisions. These METTL3-deficient CD4 + T cells also showed defects in differentiation into T FH cells and exhibited elevated apoptosis. Further, METTL3 deficiency also resulted in a decreased expression of T FH -defining genes in these nascent T FH cells. Strikingly, the abundances of Tcf7 and Bcl6 mRNAs, both essential for the early commitment of T FH cells [41] , were profoundly decreased in early METTL3-null T FH cells. Correspondingly, the protein levels of TCF-1 and Bcl-6 were also notably reduced. These findings revealed that METTL3 is required for early T FH commitment, proliferation, and survival by maintaining the key T FH gene expression. As an RNA binding protein, METTL3 is the essential catalytic component of the conserved heterodimeric m 6 A writer complex [15] . Does METTL3-mediated T FH differentiation also directly depend on its m 6 A catalytic activity? Our results showed that forced expression of METTL3 with a mutated catalytic domain failed to rectify the defects in T FH differentiation of Mettl3 fl/fl Cd4 -Cre CD4 + T cells, while wild-type METTL3 did. We thus concluded that METTL3 promotes T FH generation in an m 6 A catalytic activity-dependent manner. Giving m 6 A methylation is essential for gene expression regulation [42] , we hence focused on the methylation status of those differentially expressed genes. The expression patterns of a series of T FH -defining genes were altered at both early and mature stages, including Tcf7 , Cxcr5 , Bcl6 , Pdcd1 , and Icos . Through m 6 A-miCLIP-SMARTer-seq, we found Tcf7 mRNA was tagged by m 6 A in the 3′ UTR, whereas the other key T FH cell regulator Bcl6 mRNA was not modified. Further study indicated that METTL3-mediated m 6 A modification regulates the stability of Tcf7 mRNA, ultimately maintains TCF-1 level. Moreover, forced expression of TCF-1 could restore the T FH differentiation in the absence of METTL3. These data collectively suggested that METTL3 directly modulates the Tcf7 expression level in an m 6 A-dependent manner to promote T FH differentiation. The functional outcome of m 6 A modification is determined by an expanding list of m 6 A reader proteins in a cell type and cellular context-dependent fashion [14] , [43] . Although early evidence demonstrated that m 6 A deposition destabilizes mRNAs, resulting in their faster decay, a recent study has reported that the insulin-like growth factor 2 mRNA binding proteins (IGF2BP1-3), as a class of distinct m 6 A readers, promote m 6 A-modified mRNA stability and translation [20] . Similarly, a more recent study reported Prrc2a as a novel m 6 A reader that regulates oligodendrocyte specification and myelination by stabilizing target mRNA [44] . Our data also indicated m 6 A modification in the 3′ UTR of Tcf7 enhances its mRNA stability to promote T FH differentiation. However, the currently known IGF2BPs family readers are expressed at extremely low levels to detect in CD4 + T cells (Supplementary Fig. 8 ), implying the possibility of other unidentified proteins might be responsible for deciphering the m 6 A-modified transcripts in T FH cells. Therefore, it will be of great interest to identify new RNA-binding proteins virtually involved in T FH cells via post-transcriptional networks in future studies. In METTL3-deficient cells, destabilization of Tcf7 mRNA impacted T FH cells at least in two major aspects. The first aspect is that loss of TCF-1 expression results in massive apoptosis in T cell [45] , which is coordinated with the decreased T FH cell numbers in the absence of METTL3. The other point lies in that TCF-1 directly regulates Bcl6 mRNA expression [11] , [12] , [13] , and two of them thus collectively affect T FH differentiation. This post-transcriptional regulation of Tcf7 mRNA represents a distinct mechanism that drives T FH differentiation. It should be noted that other post-transcriptional regulators such as RNA-binding proteins and miRNAs also contribute to modulating T FH differentiation program [46] , [47] , [48] . Hence, exploring T FH fate determination on the layer of post-transcriptional level might be a fruitful effort in future investigations. A recent study referred that induced GAPDH protein by VHL deficiency reduced Icos expression through METTL3/METTL14-catalyzed m 6 A modification on Icos mRNA, implying that elevated m 6 A modification on Icos mRNA in VHL-deficient cells decreases Icos expression which is associated with attenuated T FH differentiation [49] . By analyzing high-throughput data, we also observed m 6 A modification in the 3′ UTR of Icos mRNA, and the m 6 A level on Icos mRNA was decreased in the absence of METTL3. However, we found both the mRNA and protein level of ICOS were blunted in METTL3-deficient T FH cells, indicating that loss of m 6 A modification impairs Icos expression. In addition, Zhu et al. reported that knockdown of METTL3 expression with short hairpin RNA (shRNA) in CD4 + T cells could promote T FH differentiation [49] , which differs in phenotypes from our genetic knockdown mice model. The varies may be contributed by the distinct experimental approaches and the divergent viewpoints from two studies also reflect the complex regulatory mechanism of m 6 A modification, which needs to be further disclosed. In summary, our study uncovers a critical role of METTL3-dependent m 6 A methylation in directing T FH lineage differentiation. Conditional ablation of m 6 A ‘writer’ METTL3 in CD4 + T cells intrinsically impaired the T FH differentiation, proliferation, and survival. Consequently, the GC reactions were significantly compromised in METTL3-deficient mice in response to acute viral infection. Our data indicated that METTL3 directs m 6 A modification in 3′ UTR of Tcf7 mRNA to stabilize the transcript and hence sustain TCF-1 protein expression (Fig. 8 ). Thus, m 6 A functions as an important modulator of the METTL3-TCF-1 axis to initiate and secure the differentiation of T FH cells post-transcriptionally. Fig. 8: Proposed model for m 6 A modification in promoting T FH differentiation. During acute infection, METTL3-sufficient CD4 + T cells were activated. With m 6 A machinery, Tcf7 mRNA was m 6 A modified and stabilized, allowing normal production of TCF-1 protein. TCF-1 in turn regulates expressions of T FH cell regulators, which ultimately program T FH commitment, proliferation, survival, and functional maturation. Full size image Mice Mettl3 fl/fl mice were kindly provided by Drs. Qi Zhou and Wei Li (Institute of Zoology, Chinese Academy of Sciences). SMARTA mice [50] (expressing MHC II I-A b -restricted TCR specific for LCMV glycoprotein amino acids 66–77) were generously provided by Dr. Rafi Ahmed (Emory University). Cd4 -Cre, ER T2 -Cre, and C57BL/6J (CD45.2 and CD45.1) mice were purchased from the Jackson Laboratory. All mouse strains used in this study are on a fully C57BL/6J background. All mice were kept in group housing (3–5 mice per cage) in a specific pathogen-free facility with controlled environmental conditions of humidity (50 ± 10%), lighting (a 12-h light/dark cycle), and temperature (21 ± 1 °C) at China Agricultural University. All animal experiments were performed in accordance with the protocol of the Institutional Animal Care and Use Committee of China Agricultural University. LCMV infection LCMV-Armstrong strain was grown in BHK-21 cells and titers were determined as described before [51] . Mettl3 fl/fl Cd4 -Cre mice and their wild-type littermates were intraperitoneally infected with 2 × 10 5 plaque-forming units (pfu) LCMV-Armstrong strain. In adoptive transfer experiments, recipient mice were infected 1 day after cell transfer. For bone marrow chimeric mice, LCMV infection was performed after 8 weeks reconstitution. Immunization Mettl3 fl/fl Cd4 -Cre mice and their wild-type littermates were intraperitoneally immunized with 100 μg of KLH (Sigma-Aldrich) emulsified in CFA (Sigma-Aldrich). Eight days later, splenic T cells were analyzed. Flow cytometry and antibodies Single-cell suspensions of spleens were used for flow cytometry analysis or cell sorting. Surface staining was performed in PBS containing 1% FBS. The antibodies and reagents used for flow cytometry staining are listed as: anti-CD19 (1D3; 1:100), anti-CD25 (PC61.5; 1:100), anti-CD4 (RM4-5; 1:100), anti-CD44 (IM7; 1:100), anti-CD45.1 (A20; 1:100), anti-CD45.2 (104; 1:100), anti-CD62L (MEL-14; 1:100), anti-CD69 (H1.2F3; 1:100), anti-CD8a (53-6.7; 1:100), anti-B220 (RA3-6B2; 1:100), anti-GITR (DTA-1; 1:100), anti-GL7 (GL7; 1:100), anti-PD-1 (J43; 1:100), anti-TCR Vα2 (B20.1; 1:100) (from Thermo Fisher Scientific); anti-CD138 (281-2; 1:100), anti-Fas (Jo2; 1:100) (from BD Biosciences); anti-SLAM (TC15-12F12.2; 1:100), anti-ICOS (C398.4A; 1:100) (from BioLegend), and peanut agglutinin (PNA; Cat. no. FL-1071; 1:500; Vector laboratories). CXCR5 staining was performed with a three steps staining protocol as described before [52] . Briefly, single-cell suspensions were first stained with purified anti-CXCR5 (2G8; 1:100; BD Biosciences) for 1 h, followed by biotin-conjugated goat anti-rat IgG (Cat. no. 111-066-144; 1:1,000; Jackson ImmunoResearch) for 30 min, and then by APC-eFluor 780-, or eFluor 450-labeled streptavidin (1:500; Thermo Fisher Scientific) at 4 °C for 30 min in PBS supplemented with 2% normal mouse serum (Cat. no. 015-000-120; Jackson ImmunoResearch), 2% FCS, and 0.5% BSA. For detection of cytokines, the splenocytes from KLH-immunized mice were cultured in vitro for 5 h in 2 μg/mL of PMA (Cat. no. P8139; Sigma-Aldrich), 2 μg/mL of Ionomycin (Cat. no. I0634; Sigma-Aldrich), GolgiStop (BD Biosciences), and GolgiPlug (BD Biosciences). Intracellular staining for cytokines was performed with monoclonal antibody against to IL-4 (11B11; 1:100; Thermo Fisher Scientific) and IL-17a (TC11-18H10; 1:100; BD Biosciences), using the Fixation/Permeabilization buffer kit (BD Biosciences). For intracellular staining of Bcl-6 (K112-91; 1:20; BD Biosciences), Foxp3 (FJK-16s; 1:100; Thermo Fisher Scientific), GATA3 (TWAJ; 1:100; Thermo Fisher Scientific), RORγt (AFKJS-9; 1:100; Thermo Fisher Scientific), TCF-1 (C63D9; 1:100; Cell Signaling Technology), and METTL3 (Cat. no. ab195352; 1:100; Abcam), Foxp3/Transcription Factor Staining Buffer Set (Thermo Fisher Scientific) was used following the manufacturer’s instructions. Active Caspase-3 was detected using the CaspGLOW™ Fluorescein Active Caspase-3 Staining Kit (Cat. no. 88-7004-42; 1:200; Thermo Fisher Scientific). All data were collected on a FACSVerse (BD Biosciences) with FACSSuite software (v1.0.5) or an LSRFortessa (BD Biosciences) with FACSDiva software (v8.0.2) and were analyzed with FlowJo software (v10; Treestar). The gating strategies for flow cytometry data analysis are illustrated in Supplementary Fig. 7 . Adoptive transfer To characterization of cell division at early T FH differentiation, SMARTA CD4 + T cells were labeled with 5 μM of CTV (Invitrogen), and 2 × 10 6 of labeled Vα2 + SMARTA CD4 + cells were transferred followed by intravenously infected with 2 × 10 6 pfu of LCMV-Armstrong. To investigate the intrinsic effects with adoptive transfer model, 5 × 10 6 wild-type SMARTA cells were transferred into Ctrl and Mettl3 fl/fl Cd4 -Cre host mice, followed by 2 × 10 5 pfu LCMV-Armstrong infection intraperitoneally. Bone marrow chimeric mice To generate bone marrow chimeric mice, lethally irradiated B6.SJL (CD45.1 + ) mice were transferred intravenously with a 1:1 mixture of 2.5 × 10 6 Mettl3 fl/fl Cd4 -Cre (CD45.2 + ) and 2.5 × 10 6 B6.SJL (CD45.1 + ) bone marrow cells. After 8 weeks reconstitution, recipient mice were infected with LCMV-Armstrong strain. ELISA Analysis of the LCMV-specific antibody in serum was performed as previously described [53] . Briefly, lysates of LCMV-infected BHK-21 cells were used as substrate and LCMV-specific antibody (IgG) was titrated in serial dilutions of serum using HPR-conjugated goat-anti mouse IgG antibodies (Cat. no. A90-131P-39; 1:5,000; Bethyl laboratories). Immunofluorescence staining Tissue specimens submerged in OCT compound were quickly frozen in liquid nitrogen and cut into 10 μm thickness. Frozen tissue sections were then fixed in cold acetone for 30 min at −20 °C, blocked with 1% BSA and Fc-blocker (2.4G2; 1:100; BD Biosciences) in PBS. The tissue sections were then stained with biotinylated PNA (Cat. no. BA-0074; 1:20; Vector laboratories), followed by staining with BV510-labeled anti-CD4 (RM4-5; 1:100; BD Biosciences), APC-labeled anti-IgD (11-26c; 1:100; Thermo Fisher Scientific), and AF488-conjugated streptavidin (1:500; Invitrogen). Then the slides were washed at least three times with PBS. Coverslips were mounted on slides using an antifade kit (Beyotime Biotechnology) and then examined using an Andor Dragonfly confocal microscope. The images were processed with Imaris (v8.1; Bitplane) and Image J (v1.52 g; NIH). Retroviral vectors, transduction, and cell transfer Tcf7 (full-length CDS region of P45 isoform without 3′ UTR region [39] ) and Mettl3 (wild-type and catalytic domain dead) coding sequences were amplified and cloned into the pMIG-R1 vector (MSCV-IRES-GFP). Retrovirus was packaged by transfection of HEK293T cells (Cat. no. CRL-3216; ATCC) with the retroviral vectors along with pCL eco plasmid. SMARTA cells were activated in vivo by injection of 200 μg of LCMV GP61-80 (GLNGPDIYKGVYQFKSVEFD) peptide into Mettl3 fl/fl Cd4 -Cre SMARTA mice or their littermate wild-type transgenic mice. After 16~18 h, activated SMARTA cells were isolated, purified, and ‘spin-infected’ for 120 min at 37 °C by centrifugation (1000 × g ) with freshly harvested retroviral supernatants supplemented with 8 μg/mL of polybrene (Sigma-Aldrich), then cultured overnight in the presence of 20 ng/mL of IL-2 (Peprotech), and 250 nM of LCMV GP61-80. The spinofection was repeated the next day, and a total of 0.5~1 × 10 6 retroviral infected SMARTA CD4 + T cells were then adoptively transferred into recipient mice, followed by infection of the hosts with 2 × 10 5 pfu LCMV-Armstrong within 24 h. RNA-seq and data analysis For isolation of T H 1 cells and T FH cells, splenocytes from Mettl3 fl/fl Cd4 -Cre mice and their control littermates on day 8 post viral infection were subjected to depletion of cells positive for lineages markers by using biotin-conjugated antibodies (anti-B220 (RA3-6B2; 1:100), anti-CD8 (53-6.7; 1:100), anti-Gr.1 (RB6-8C5; 1:100), anti-CD11b (M1/70; 1:100), anti-CD11c (N418; 1:100), anti-TER119 (TER-119; 1:100), and anti-CD49b (DX5; 1:100); all from Thermo Fisher Scientific) coupled to Dynabeads M-280 Streptavidin (Invitrogen), followed by surface stained. CD44 + SLAM hi T H 1 cells and CD44 + SLAM lo T FH cells were sorted with a FACSAria II cell sorter (BD Biosciences) with FACSDiva software (v7.0) and subsequently lysed with TRIzol Reagent (Life technologies). Total RNAs were extracted and then subjected to Annoroad (Beijing, China) for library construction and RNA sequencing. The qualities of clean reads were assessed by FastQC (v0.11.5). Then the reads were mapped to mouse genome mm10 (version M17) using TopHat (v2.1.1). The read counts of all genes were estimated by HTseq (v0.6.1) and differentially expressed genes were identified by DESeq2 (v1.18.1). TPM, FPKM, and RPKM were calculated, and upregulated or downregulated genes in Mettl3 fl/fl Cd4 -Cre T FH or T H 1 cells were identified by expression changes ≥ 2-fold and FDR < 0.01. Quantitative RT-PCR Total RNAs were extracted from sorted cells using RNeasy Mini Kit (Qiagen) followed by cDNA synthesis with FastQuant RT Kit (Tiangen). Quantitative RT-PCR was carried out with SuperReal PreMix Plus SYBR Green (Tiangen) on a CFX96 Connect TM Real-Time System (Bio-Rad). Results were processed by Microsoft Excel and then were normalized to the expression of Hprt1 transcripts. Fold differences in expression levels were calculated according to the 2 −ΔΔCT method. 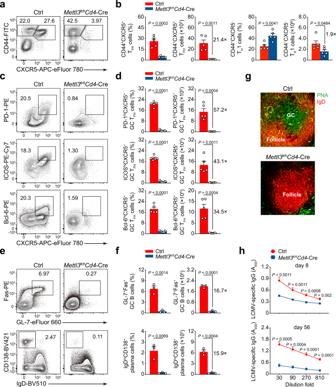Fig. 1: Conditional ablation of METTL3 impairs TFHdifferentiation and GC responses. a,bFlow cytometry analysis of CD44+CXCR5+TFHcells and CD44+CXCR5–TH1 cells, gated on splenic CD4+T cells from Ctrl andMettl3fl/flCd4-Cre mice on day 8 post infection (8dpi). Summary of the frequency and cell numbers of indicated cell subsets are shown inb(n= 5 per group).c,dFlow cytometry analysis of PD-1hiCXCR5+GC TFHcells (top panel), ICOShiCXCR5+GC TFHcells (middle panel), and Bcl-6hiCXCR5+GC TFHcells (bottom panel), gated on splenic CD44hiCD62LloCD4+T cells from Ctrl andMettl3fl/flCd4-Cre mice on 8dpi. Summary of the frequency and cell numbers of indicated cell subsets are shown ind(n= 5 per group).e,fFlow cytometry analysis of splenic GL-7+Fas+GC B cells (top panel) and IgDloCD138+plasma cells (bottom panel) on 8dpi. Summary of the frequency and cell numbers of GC B cells and plasma cells are shown inf(n= 3 per group).gImmunofluorescent staining of spleens from Ctrl andMettl3fl/flCd4-Cre on 8dpi. Green: PNA; Red: IgD; scale bar: 10 μm.hAnalysis of LCMV-specific IgG concentration in serum on 8dpi(top) and on 56dpi(bottom) by ELISA (day 8:n= 12 for Ctrl group,n= 10 forMettl3fl/flCd4-Cre group; day 56:n= 5 per group). Data are representative of at least three independent experiments. Error bars indicate standard error of the mean.Pvalue was calculated by unpaired two-tailed Student’sttest. All primers used are listed in Supplementary Table 1 . Gene set enrichment analysis GSEA was performed with GSEA desktop software (v4.1.0) from the Broad Institute. The T FH gene set [11] , GC T FH gene set [11] , T H 1 gene set [12] , T H 2 gene set [34] , T H 17 gene set [35] , and Treg gene set [34] have been described before. The ‘TCF1-activated genes in T FH cells’ gene set contains 569 genes that are downregulated by ≥1.5-fold in Tcf7 fl/fl Cd4 -Cre T FH cells; The ‘TCF1-suppressed genes in T FH cells’ gene set contains 513 genes that are upregulated by ≥1.5-fold in Tcf7 fl/fl Cd4 -Cre T FH cells (GSE65693). Luciferase reporter assay Tcf7 3′ UTR segment (~200 nt) was amplified from a mouse double-positive (DP) thymocytes cDNA library by PCR and inserted into the pGL4.23 vector (Promega) by using XbaI and FseI restriction sites. The Tcf7 3′ UTR mutation plasmids were generations from site-directed mutagenesis. All plasmids and mutations were verified by sequencing. HEK293T cells were seeded into 24-well plates in triplicate to allow 80% confluency in the next day. A total of 200 ng of reporter plasmids (Fluc) and 20 ng of Renilla luciferase (Rluc) control plasmids (pRL-TK) were co-transfected using Lipofectamine 2000 reagent (Invitrogen) under METTL3 overexpressing. Fluc and Rluc activities were measured 24 h later with the Dual-Luciferase Reporter Assay System (Promega) according to the manufacturer’s instructions. The relative luciferase activity was calculated by dividing Fluc by Rluc and normalized to pGL4.23 empty vector for each assay. RNA decay assay CD4 + T cells were purified from Mettl3 fl/fl ER T2 -Cre mice and their control wild-type mice as described above. 5 × 10 5 purified CD4 + T cells in RPMI 1640 medium supplemented with 10% fetal bovine serum, 20 ng/mL of IL-2, 10 ng/mL of IL-7, and 5 μM of 4-Hydroxytamoxifen (Sigma-Aldrich) were seeded into 48-well plates. After 48 h, actinomycin D (MedChemExpress) was added to a final concentration of 5 μM, and cells were harvested at t = 0, 1, 2 h after actinomycin D treatment. Total RNAs were extracted and subjected to RT-qPCR analysis. Results were processed by Microsoft Excel and then normalized to the expression of Gapdh transcript. Fold differences in expression levels were calculated according to the 2 –ΔΔCT method. All primers used are listed in Supplementary Table 1 . 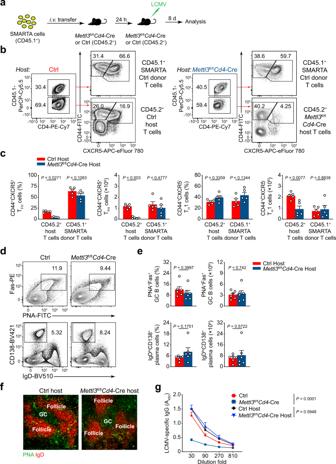Fig. 2: METTL3 intrinsically controls TFHdifferentiation and GC responses. aScheme of adoptive transfer model. 5 × 106CD45.1+SMARTA cells were adoptively transferred into CD45.2+Mettl3fl/flCd4-Cre mice or Ctrl host mice, followed by LCMV-Armstrong infection within 24 h.b,cFlow cytometry analysis of CD45.1+SMARTA or CD45.2+host T cell-derived CD44+CXCR5+TFHand CD44+CXCR5–TH1 cells, gated on splenic CD4+T cells from host mice on day 8 post viral infection. Frequency and numbers of CD44+CXCR5+TFHcells and CD44+CXCR5–TH1 cells are shown inc(n= 5 per group).d,eFlow cytometry analysis of splenic PNA+Fas+GC B cells (top panel) and IgDloCD138+plasma cells (bottom panel) from host mice on 8dpi. Summary of the frequency and cell numbers of GC B cells and plasma cells are shown ine(n= 6 per group).fImmunofluorescent staining of spleens from Ctrl orMettl3fl/flCd4-Cre host mice on 8dpi. Green: PNA; Red: IgD; scale bar: 10 μm.gAnalysis of LCMV-specific IgG concentration in serum on 8dpiby ELISA (n= 5 for Ctrl group,n= 5 forMettl3fl/flCd4-Cre group,n= 6 for Ctrl host group,n= 6 forMettl3fl/flCd4-Cre host group). Data are representative of at least three independent experiments. Error bars indicate standard error of the mean.Pvalue was calculated by unpaired two-tailed Student’sttest (e) or two-way ANOVA coupled with multiple comparisons (c,g). m 6 A-miCLIP-SMARTer-seq and data processing Total RNAs from CD4 + SMARTA cells sorted from LCMV GP61-80-primed Mettl3 fl/fl Cd4 -Cre SMARTA or Ctrl SMARTA mice were extracted with TRIzol Reagent (Life Technologies). mRNAs were further isolated from total RNAs using Dynabeads mRNA purification kit (Ambion). The procedures of m 6 A-miCLIP-SMARTer-seq were according to the previously reported methods with some modifications [54] . 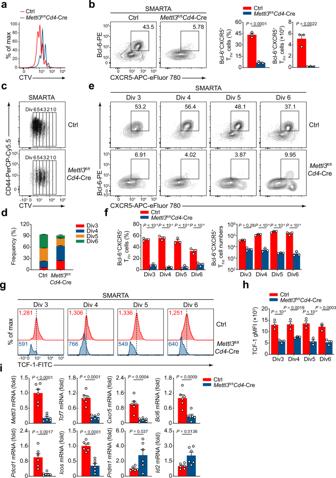Fig. 3: METTL3 is indispensable for the initiation of TFHdevelopment. aFlow cytometry analysis of cells from the wild-type recipient mice (CD45.1+) given adoptive transfer of naive CTV-labeled Ctrl orMettl3fl/flCd4-Cre SMARTA cells, followed by LCMV-Armstrong infection and analysis 3 days later as CTV dilution by the transferred cells.bFlow cytometry analysis of Bcl-6+CXCR5+TFHcells gated on SMARTA CD4+T cells from recipient mice as ina. Summary of the frequency and cell numbers of TFHcells are shown on the right (n= 3 per group).c,dFlow cytometry analysis of different cell divisions gated on SMARTA CD4+T cells from recipient mice as ina. The frequency of third to sixth divisions is summarized ind(n= 3 per group).e,fContour plots display Bcl-6+CXCR5+TFHcells in indicated divisions, among SMARTA cells from recipient mice as ina. Summary of the frequency and cell numbers of TFHcells in indicated divisions are shown inf(n= 3 per group).g,hFlow cytometry analysis of the expression of TCF-1 in CXCR5+cells in indicated divisions gated on SMARTA CD4+T cells from recipient mice as ina. Quantification of geometric mean fluorescence intensity (gMFI) of TCF-1 in indicated divisions is shown inh(n= 3 per group).iQuantitative RT-PCR analysis of mRNA abundance of TFHcell-related genes in CD25–CXCR5+TFHcells from recipient mice as ina, relative expression was normalized to Ctrl cells (n= 6 per group). Data are representative of two independent experiments. Error bars indicate standard error of the mean.Pvalue was calculated by unpaired two-tailed Student’sttest (b,i) or two-way ANOVA coupled with multiple comparisons (f,h). Briefly, 100 ng of mRNAs were fragmented to ~100 nt by using the fragmentation reagent (Life Technologies) and incubated with 5 μg of specific antibody against m 6 A (Abcam) in 500 μL of immunoprecipitation buffer (50 mM Tris-HCl (pH 7.4), 100 mM NaCl, 0.05% NP-40) with gentle rotation at 4 °C for 2 h. The mixture was then transferred into a clear flat-bottom 96-well plate (Corning) on ice and irradiated three times with 0.15 J/cm −2 at 254 nm in a CL-1000 Ultraviolet Crosslinker (UVP). The irradiated mixture was then transferred to a new tube and incubated with 50 μL of pre-washed Dynabeads Protein A (Life Technologies) at 4 °C for 2 h. After extensive washing twice with high-salt wash buffer (50 mM Tris-HCl (pH 7.4), 1 M NaCl, 1 mM EDTA, 1% NP-40, 0.1% SDS) and twice with immunoprecipitation buffer, the mixture on beads was subjected to dephosphorylation with T4 PNK (NEB) for 20 min at 37 °C. After extensive washing, the RNA was eluted from the beads by proteinase K (Sigma-Aldrich) digestion at 55 °C for 1 h, followed by phenol-chloroform extraction and ethanol precipitation. The purified RNA was subjected to library construction using a SMARTer smRNA-Seq Kit for Illumina (Clontech Laboratories) according to the manufacturer’s instructions. 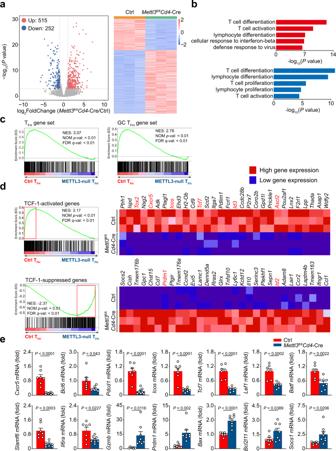Fig. 4: Alternation of transcriptional profiles in METTL3-null TFHcells. aVolcano map depicting genes upregulated (red) or downregulated (blue) 2-fold or more in TFHcells on 8dpi. Heatmap of differentially expressed genes is shown on the right.bGene Ontology (GO) terms of the differentially expressed genes inMettl3fl/flCd4-Cre TFHcells compared with Ctrl TFHcells (Upregulated: top panel; Downregulated: bottom panel).cGene set enrichment analysis (GSEA) of TFHand GC TFHgene set inMettl3fl/flCd4-Cre TFHcells relative to expression in Ctrl TFHcells as ina.dGSEA analysis of “TCF-1-activated genes in TFHcells” and “TCF-1-suppressed genes in TFHcells” (GSE65693) inMettl3fl/flCd4-Cre TFHcells relative to expression in Ctrl TFHcells as ina. Heatmaps representation of top 30 ranking genes in the leading edge are shown, respectively.eQuantitative RT-PCR analysis of selected interested genes ina, relative expression was normalized to that in Ctrl TFHcells (n= 7 for Ctrl group,n= 8 forMettl3fl/flCd4-Cre group exceptBcl6gene (n= 7 per group)). Data are from one experiment with triplicates (a–d) or pooled from two experiments (e). Error bars indicate standard error of the mean.Pvalue was calculated by unpaired two-tailed Student’sttest (e). Sequencing was carried out on an Illumina X-ten platform. m 6 A-miCLIP-SMARTer-seq data (paired-end) were analyzed as previously described [55] . Adapter sequences at the 3′ ends were removed first. R2 reads were then transformed to reverse complementary sequences and merged with R1 reads. PolyA tails from the library were trimmed by Cutadapt (v1.17) and fastq2collapse (v1.1.3) was used to remove duplicated reads; afterward, the barcodes of reads were removed. 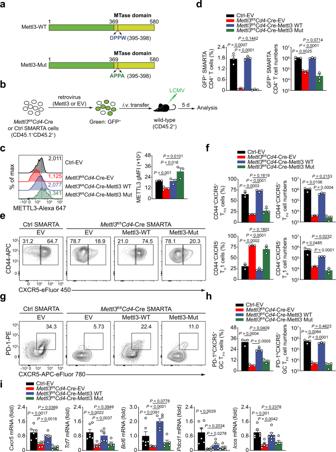Fig. 5: METTL3 promotes TFHdifferentiation in an m6A catalytic activity-dependent manner. aGraphic representation of the wild-type (Mettl3-WT) and catalytic domain dead (Mettl3-Mut; DPPW to APPA) METTL3 constructs.bScheme of retrovirus transduction experiment. SMARTA cells were transduced with indicated structures by using a retrovirus transduction system. Then, the transduced cells were adoptively transferred into congenic CD45.2+wild-type mice followed by LCMV-Armstrong infection, and analyzed on day 5 post viral infection.cFlow cytometry analysis of METTL3 gMFI in GFP+CD4+SMARTA cells from recipient mice. Quantitation of METTL3 gMFI is shown on the right (n= 3 per group).dSummary of the frequency and cell numbers of retrovirus-transduced SMARTA CD4+T cells in host mice (n= 3 per group).e,fFlow cytometry analysis of CD44+CXCR5+TFHpopulations and CD44+CXCR5–TH1 subsets gated on SMARTA GFP+CD4+T cells from host mice adoptively transferred with empty vector (EV), Mettl3-WT, or Mettl3-Mut retrovirus-introduced SMARTA cells. Summary of the frequency and cell numbers of TFHcells and TH1 cells are shown inf(n= 3 per group).g,hFlow cytometry analysis of PD-1hiCXCR5+GC TFHpopulations gated on SMARTA GFP+CD4+T cells from host mice adoptively transferred with EV, Mettl3-WT, or Mettl3-Mut retrovirus-introduced SMARTA cells. Summary of the frequency and cell numbers of GC TFHcells are shown inh(n= 3 per group).iQuantitative RT-PCR analysis of mRNA abundance of TFHcell-related genes in CD44+CXCR5+TFHcells ectopically expressed with EV, Mettl3-WT, or Mettl3-Mut, relative expression was normalized to Ctrl cells transduced with EV retrovirus (n= 6 for Ctrl EV,Mettl3fl/flCd4-Cre-EV, andMettl3fl/flCd4-Cre-Mettl3 WT group;n= 5 forMettl3fl/flCd4-Cre-Mettl3 Mut group). Data are representative of two independent experiments. Error bars indicate standard error of the mean.Pvalue was calculated by one-way ANOVA, followed by unpaired two-tailed Student’sttest for indicated pairwise comparisons. Low-quality bases were discarded, and only reads longer than 18 nt were retained. The remaining reads were mapped to the reference genome (mm10) using BWA (v0.7.17) with the parameter: -n 0.06. The mutation information was extracted and PCR duplicates according to BWA’s results were removed separately by parseAlignment.pl (–map-qual 1 –min-len 18) and tag2collapse.pl (-EM 30 –seq-error-model alignment). CIMS.pl was used to calculate the coverage ( n ) of the mutation site and transition number ( m ). Mutation sites with parameters, m ≥ 3, k / m ≥ 0.01, and k / m ≤ 0.5, were kept. The remaining sites within the RRACH motif sequence were considered as m 6 A. m 6 A-RIP-qPCR Purified mRNAs of CD4 + SMARTA cells sorted from Mettl3 fl/fl Cd4 -Cre SMARTA or Ctrl SMARTA mice were prepared and fragmented into ~100 nt by RNA fragmentation reagents (Life Technologies). Immunoprecipitation was performed using anti-m 6 A antibody (Abcam) as described above. The enrichment of m 6 A was measured with quantitative RT-PCR. Primers for m 6 A-RIP-qPCR are listed in Supplementary Table 1 . RIP-qPCR 5 × 10 6 CD4 + SMARTA T cells were isolated and lysed with 1 mL cell lysis buffer (150 mM KCl, 10 mM HEPES (pH 7.6), 2 mM EDTA, 0.5% NP-40, 0.5 mM DTT, 1:100 proteinase inhibitor cocktail, and 0.4 U/µL RNasin) at 4 °C for 30 min. After centrifugation, the supernatant (10% of which was kept as input) was subjected to RNA immunoprecipitation with anti-METTL3 (Abcam) coupled with Dynabeads Protein A (Life Technologies). RNA was isolated from the beads and input samples for RT-qPCR. Primers for RIP-qPCR are listed in Supplementary Table 1 . 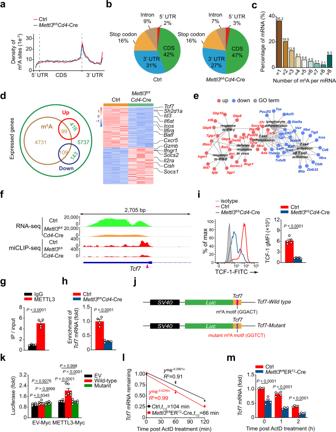Fig. 6: m6A modifiesTcf7mRNA to control its stability. aMetagene profiles of m6A site distribution along a normalized transcript containing three rescaled non-overlapping segments: 5′ UTR, CDS, and 3′ UTR in Ctrl andMettl3fl/flCd4-Cre SMARTA CD4+T cells.bPie chart showing the distribution of m6A sites in five regions of Ctrl andMettl3fl/flCd4-Cre SMARTA CD4+T cells.cBar chart depicting percentage of mRNAs with different internal m6A abundance.dVenn diagram showing the overlapping differentially expressed genes from RNA-seq and m6A-modified transcripts from m6A-miCLIP-SMARTer-seq. Heatmap of 208 differentially expressed genes with m6A modification is shown on the right.eRepresentative GO terms of the biological process categories enriched in differentially expressed transcripts with m6A peaks (Red: upregulated genes; blue: downregulated genes; gray: GO terms).fIntegrative Genomics Viewer (IGV) tracks displaying RNA-seq (top panel) and m6A-miCLIP-SMARTer-seq (bottom panel) reads distribution ofTcf7gene. The high-confidence m6A site is marked as a triangle.gRIP-qPCR analysis showing enrichment of METTL3 onTcf7mRNA in SMARTA CD4+T cells. TheTcf7mRNA enrichment is presented as IP/input and normalized to IgG group (n= 4 per group).hm6A-RIP-qPCR analysis of m6A enrichment onTcf7mRNA of Ctrl andMettl3fl/flCd4-Cre SMARTA CD4+T cells (n= 4 per group).iFlow cytometry analysis of expression level of TCF-1 on TFHcells on 8dpi. Quantification of gMFI of TCF-1 is shown on the right (n= 5 per group).jConstructions of plasmids with wild-type or m6A site mutant inTcf73′ UTR.kLuciferase reporter assay. Results were normalized to the luciferase activity of cells co-transfected with the pGL4.23 empty plasmid and EV-Myc plasmid (n= 6 per group).lRNA decay assay. The half-live ofTcf7mRNA was detected by quantitative RT-PCR. The remaining mRNAs were normalized tot= 0 (n= 4 per group).mQuantitative RT-PCR analysis ofTcf7mRNA abundance as inl, relative expression was normalized tot= 0 of Ctrl cells (n= 4 per group). Data are from one experiment with duplicate (a–e) or representative of at least three independent experiments (i–h,k–m). Error bars indicate standard error of the mean.Pvalue was calculated by unpaired two-tailed Student’sttest (g–i) or two-way ANOVA coupled with multiple comparisons (k,m). 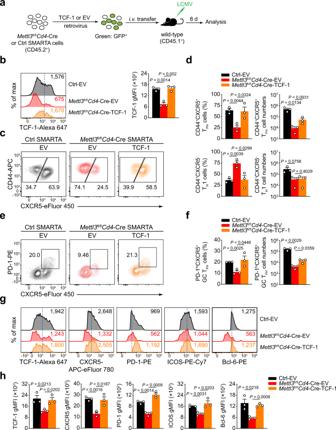Fig. 7: Enhanced TCF-1 expression rectifies defective TFHdifferentiation in METTL3-null cell. aScheme of TCF-1 rescue experiment. SMARTA cells were transduced with TCF-1 structure (full-length CDS of P45 isoform without 3′ UTR region) by using a retrovirus transduction system. Then, the transduced cells were adoptively transferred into congenic CD45.1+wild-type mice followed by LCMV-Armstrong infection, and analyzed on day 8 post viral infection.bFlow cytometry analysis of TCF-1 gMFI in SMARTA GFP+CD4+cells from recipient mice on 8dpi. Quantitation of TCF-1 gMFI is shown on the right (n= 3 per group).c,dFlow cytometry analysis of CD44+CXCR5+TFHpopulations and CD44+CXCR5–TH1 subsets gated on SMARTA GFP+CD4+T cells from different host mice adoptively transferred with empty vector (EV) or TCF-1 retrovirus-introduced SMARTA cells at 8 days post infection. Summary of the frequency and cell numbers of TFHcells and TH1 cells are shown ind(n= 3 per group).e,fFlow cytometry analysis of PD-1hiCXCR5+GC TFHpopulations gated on SMARTA GFP+CD4+T cells from different host mice adoptively transferred with EV or TCF-1 retrovirus-introduced SMARTA cells. Summary of the frequency and cell numbers of GC TFHcells are shown inf(n= 3 per group).g,hFlow cytometry analysis of gMFIs of TCF-1, CXCR5, PD-1, ICOS, and Bcl-6 on CD44+CXCR5+TFHcells transduced with EV or TCF-1 retrovirus. Quantification of the gMFIs is shown inh(n= 3 per group). Data are representative of three independent experiments. Error bars indicate standard error of the mean.Pvalue was calculated by one-way ANOVA, followed by unpaired two-tailed Student’sttest for indicated pairwise comparisons. 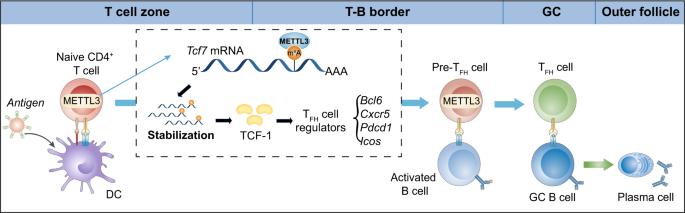Fig. 8: Proposed model for m6A modification in promoting TFHdifferentiation. During acute infection, METTL3-sufficient CD4+T cells were activated. With m6A machinery,Tcf7mRNA was m6A modified and stabilized, allowing normal production of TCF-1 protein. TCF-1 in turn regulates expressions of TFHcell regulators, which ultimately program TFHcommitment, proliferation, survival, and functional maturation. Statistical analysis Statistical analysis was performed with Prism 8.0 (GraphPad). An unpaired two-tailed Student’s t test with a 95% confidence interval, one-way ANOVA, or two-way ANOVA analysis was used to calculate P values. Reporting summary Further information on research design is available in the Nature Research Reporting Summary linked to this article.